Emi2 mediates meiotic MII arrest by competitively inhibiting the binding of Ube2S to the APC/C In vertebrates, unfertilized eggs are arrested at metaphase of meiosis II by Emi2, a direct inhibitor of the APC/C ubiquitin ligase. Two different ubiquitin-conjugating enzymes, UbcH10 and Ube2S, work with the APC/C to target APC/C substrates for degradation. However, their possible roles and regulations in unfertilized/fertilized eggs are not known. Here we use Xenopus egg extracts to show that both UbcH10 and Ube2S are required for rapid cyclin B degradation at fertilization, when APC/C binding of Ube2S, but not of UbcH10, increases several fold, coincidently with (SCF β-TrCP -dependent) Emi2 degradation. Interestingly, before fertilization, Emi2 directly inhibits APC/C–Ube2S binding via the C-terminal tail, but on fertilization, its degradation allows the binding mediated by the Ube2S C-terminal tail. Significantly, Emi2 and Ube2S bind commonly to the APC/C catalytic subunit APC10 via their similar C-terminal tails. Thus, Emi2 competitively inhibits APC/C–Ube2S binding before fertilization, while its degradation on fertilization relieves the inhibition for APC/C activation. The meiotic cell cycle consists of two successive divisions, meiosis I and meiosis II. In vertebrates, mature oocytes (or unfertilized eggs) are arrested at metaphase of meiosis II (Meta-II) by a cytostatic factor (CSF) to await fertilization [1] , [2] . CSF inhibits the anaphase-promoting complex/cyclosome (APC/C), a multisubunit E3 ubiquitin ligase [3] , thereby preventing degradation of cyclin B and, hence, exit from Meta-II (ref. 4 ). CSF consists mainly of the classical Mos-MAPK pathway [2] , [4] and Emi2 (also called Erp1), a direct inhibitor of the APC/C [5] , [6] , [7] . The Mos-MAPK pathway directly phosphorylates Emi2 and upregulates both its stability and activity, thus robustly inhibiting the APC/C [8] , [9] . Both Mos and Emi2 are degraded on fertilization, although Emi2 is re-synthesized shortly later [5] , [10] , [11] , [12] . Cyclin B degradation on fertilization, owing to Emi2 degradation and hence APC/C activation, is essential for the exit from Meta-II (ref. 13 ). Emi2 consists of an N-terminal regulatory region and a C-terminal functional region. The N-terminal region possesses signals required for the rapid, calcium-induced and SCF β-TrCP ubiquitin ligase-dependent degradation of Emi2 on fertilization [14] , [15] . On the other hand, the C-terminal region contains a destruction box (D-box), which may compete with cyclin B for APC/C binding, and a zinc-binding region (ZBR), which inhibits APC/C ubiquitin ligase activity [5] , [16] , [17] . In addition, the well-conserved C-terminal tail, termed the RL tail, directly binds to the APC/C and helps the inhibitory interactions of the D-box and the ZBR with the APC/C [18] . By recruiting PP2A-B56 phosphatase, the Mos-MAPK pathway antagonizes Emi2 inhibitory phosphorylations by cyclin B-Cdk1, which occur on both the N-terminal and C-terminal regions, including the RL tail [19] , [20] . The APC/C is a large, multisubunit E3 ubiquitin ligase that targets various cell cycle regulators, including cyclin B and securin, for 26S proteasome-dependent degradation [3] , [21] , [22] . In higher eukaryotes including vertebrates, the APC/C assembles Lys11-linked ubiquitin chains on APC/C substrates by utilizing two different E2 ubiquitin-conjugating enzymes, UbcH10 and Ube2S [22] , [23] , [24] . UbcH10 is responsible primarily for monoubiquitination (or initiation of polyubiquitination) of APC/C substrates [24] , [25] , whereas Ube2S catalyses ubiquitin chain elongation (or polyubiquitination) of the monoubiquitinated APC/C substrates [26] , [27] , [28] . Co-depletion of UbcH10 and Ube2S abrogates Lys11-linked polyubiquitination of APC/C substrates, stabilizing APC/C substrates and resulting in severe mitotic delay in human cells [27] , [29] . However, Ube2S may be required for normal mitosis only in a subset of cell types, although it may be important for recovery from the spindle checkpoint in human cells [26] , [27] . Indeed, a recent study showed that UbcH10 is sufficient for cyclin B1 degradation in mitotically arrested Xenopus egg extracts because, in cyclin B1, UbcH10 can catalyse multiple monoubiquitination (monoubiquitination at multiple sites) instead of polyubiquitination, which is catalysed by Ube2S [30] . Thus, it will be interesting to know whether Ube2S plays any role in cyclin B degradation in any other biological systems, such as fertilization of vertebrate eggs, in which cyclin B degradation plays an essential role as described above. In this study, we examined whether Ube2S plays a role in cyclin B (B1 and B2) degradation and undergoes any regulation, on release from Meta-II (CSF) arrest of Xenopus eggs (or egg extracts). Our results show that Ube2S is required for both cyclin B1 and B2 degradation on CSF release, and that Emi2 directly inhibits APC/C–Ube2S binding via the RL tail during CSF arrest, while its degradation on CSF release allows the binding for APC/C activation. Furthermore, we demonstrate that Emi2 and Ube2S bind commonly to the APC/C catalytic core subunit APC10 via their similar C-terminal tails. Thus, our results reveal that Emi2 regulation of APC/C–Ube2S binding plays a physiologically important role during CSF arrest and release (or fertilization) of Xenopus eggs. At the nearly final step of this work, Wang and Kirschner [31] reported that the C-terminal tail of Emi1, a somatic paralog of Emi2, can competitively inhibit APC/C–Ube2S binding in vitro , and that both Emi1 and Ube2S bind to the APC/C cullin subunit APC2. Ube2S is required for cyclin B degradation on CSF release UbcH10, a ubiquitination-initiating E2 enzyme, and Ube2S, a ubiquitin chain-elongating E2 enzyme, both work with the APC/C E3 ubiquitin ligase to form Lys11-linked chains on APC/C substrates [23] , [32] . Reportedly, multiple monoubiquitination by UbcH10 is sufficient for APC/C-dependent degradation of cyclin B1, which carries numerous ubiquitinatable Lys residues in the N terminus [30] . We initially asked whether UbcH10 and Ube2S undergo any regulation on expression levels during CSF arrest and release of Xenopus eggs, and whether they play a role in the degradation of cyclin B1 and B2 on CSF release. To this end, we raised, in rabbits, antibodies specific to Xenopus UbcH10 and Ube2S proteins, identified these E2 enzymes in unfertilized egg extracts (CSF extracts) and estimated their concentrations to be 180 nM and 220 nM, respectively ( Fig. 1a ). On calcium addition to CSF extracts (which mimics fertilization, releasing Meta-II or CSF arrest), the APC/C inhibitor Emi2, cyclin B1 and B2 were degraded, in this order, very rapidly or within minutes (Emi2 degradation is dependent on SCF β-TrCP but not the APC/C), as previously shown [8] , [15] , but both UbcH10 and Ube2S, like APC/C core subunits Cdc27 and APC8 and its coactivator Cdc20, were very stable at least for 30 min ( Fig. 1b ). Furthermore, whereas many other proteins such as Emi2 and Cdc27 showed gel mobility shifts due to phosphorylation/dephosphorylation, neither UbcH10 nor Ube2S showed such mobility shifts ( Fig. 1b ). Thus, UbcH10 and Ube2S are both unlikely to be regulated on the level of expression or phosphorylation during CSF arrest and release. 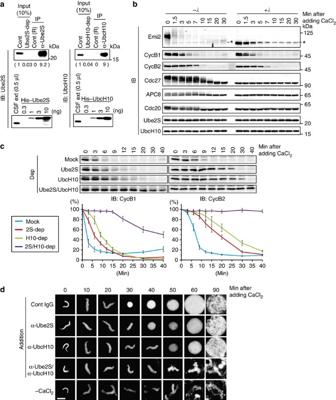Figure 1: Ube2S is required for the degradation of cyclin B1 and B2 on CSF release. (a) UbcH10 and Ube2S proteins were identified by immunoprecipitation (IP) and immunoblotting (IB) of CSF extracts, while their concentrations in CSF extracts were determined by using bacterially produced His6-tagged UbcH10 and Ube2S proteins as standards. For input (10%), both control and Ube2S- or UbcH10-immunodepleted extracts were used. Intensities of the blot bands, quantitated using Science Lab 2003 Image Gauge (FUJIFILM), are shown in relative amounts in parentheses. dep, immunodepleted; Cont (R), control rabbit IgG; α-, antibody. (b) After calcium addition, CSF extracts were collected at the indicated times, treated or not treated with λ phosphatase (λ) and immunoblotted for the indicated proteins. Note that Emi2 and cyclin B1 start to be re-synthesized 20–30 min after calcium addition. Asterisk, non-Emi2 background protein. (c) CSF extracts immunodepleted (Dep) of endogenous UbcH10 and/or Ube2S were added with calcium, collected at the indicated times and immunoblotted for cyclin B1 and B2. Kinetics graphs summarizing four independent experiments are also shown (with mean±s.d.), with the levels of cyclin B1 or B2 at time 0 in the respective immunodepleted extracts being all set at 100. (d) CSF extracts were incubated with anti-UbcH10 and/or anti-Ube2S antibodies for 15 min, further incubated with demembranated sperm nuclei for 5 min, added with calcium and collected at the indicated times for nuclear staining with Hoechst 33342. Scale bar, 10 μm. Figure 1: Ube2S is required for the degradation of cyclin B1 and B2 on CSF release. ( a ) UbcH10 and Ube2S proteins were identified by immunoprecipitation (IP) and immunoblotting (IB) of CSF extracts, while their concentrations in CSF extracts were determined by using bacterially produced His 6 -tagged UbcH10 and Ube2S proteins as standards. For input (10%), both control and Ube2S- or UbcH10-immunodepleted extracts were used. Intensities of the blot bands, quantitated using Science Lab 2003 Image Gauge (FUJIFILM), are shown in relative amounts in parentheses. dep, immunodepleted; Cont (R), control rabbit IgG; α-, antibody. ( b ) After calcium addition, CSF extracts were collected at the indicated times, treated or not treated with λ phosphatase (λ) and immunoblotted for the indicated proteins. Note that Emi2 and cyclin B1 start to be re-synthesized 20–30 min after calcium addition. Asterisk, non-Emi2 background protein. ( c ) CSF extracts immunodepleted (Dep) of endogenous UbcH10 and/or Ube2S were added with calcium, collected at the indicated times and immunoblotted for cyclin B1 and B2. Kinetics graphs summarizing four independent experiments are also shown (with mean±s.d. ), with the levels of cyclin B1 or B2 at time 0 in the respective immunodepleted extracts being all set at 100. ( d ) CSF extracts were incubated with anti-UbcH10 and/or anti-Ube2S antibodies for 15 min, further incubated with demembranated sperm nuclei for 5 min, added with calcium and collected at the indicated times for nuclear staining with Hoechst 33342. Scale bar, 10 μm. Full size image We then addressed whether UbcH10 and Ube2S were required for the degradation of cyclin B1 and B2 on CSF release. Nearly complete (>96%) immunodepletion of either UbcH10 or Ube2S from CSF extracts (see Fig. 1a and Methods) had no detectable effects on the levels of cyclin B1 and B2 during CSF arrest ( Supplementary Fig. 1a ). On CSF release, however, UbcH10 depletion delayed the degradation of cyclin B1 and B2 by ~10 min and ~25 min, respectively, as compared with mock depletion ( Fig. 1c ). Interestingly, Ube2S depletion also delayed the degradation of cyclin B1 and B2, albeit somewhat less effectively than UbcH10 depletion, and co-depletion of UbcH10 and Ube2S nearly completely inhibited the degradation of both cyclins ( Fig. 1c ). In these experiments, adding recombinant UbcH10 and/or Ube2S proteins back to the UbcH10- and/or Ube2S-depleted extracts was able to restore the delayed or inhibited degradation of cyclin B1 and B2 ( Supplementary Fig. 1b ). Furthermore, we obtained essentially the same results as these (by immunodepletion) by simply adding anti-UbcH10 and/or anti-Ube2S antibodies (which most likely worked as neutralizing antibodies) to CSF extracts ( Supplementary Fig. 1c ). Thus, these results show that, although multiple monoubiquitination by UbcH10 may be sufficient for cyclin B1 degradation in mitotically arrested Xenopus egg extracts [30] , Ube2S and UbcH10 are required for the rapid degradation of both cyclin B1 and B2 on release from meiotic CSF arrest. On CSF release, we also observed significant effects of either UbcH10 or Ube2S inhibition (by simple antibody addition) on the timing of nuclear envelope formation around the added, demembranated sperm nuclei (which occurred significantly later than cyclin B degradation) ( Fig. 1d ). Furthermore, co-inhibition of UbcH10 and Ube2S completely inhibited the nuclear envelope formation, with the sperm chromosomes undergoing rather M phase-like condensation as in calcium-untreated control extracts ( Fig. 1d ). Thus, Ube2S and UbcH10 probably play an important physiological role in calcium-induced CSF release, or fertilization, of Xenopus eggs. APC/C–Ube2S interactions increase on CSF release Given the above results, on CSF release, UbcH10 and/or Ube2S may be positively regulated on some other level(s) than expression or phosphorylation. Specifically, because APC/C activity is inhibited by Emi2 during CSF arrest, on CSF release UbcH10 and/or Ube2S might be somehow positively regulated by Emi2 degradation, possibly on the level of their interactions with the APC/C. To test this possibility, we performed co-immunoprecipitation experiments in which Cdc27 immunoprecipitates were immunoblotted for UbcH10, Ube2S or other proteins before and after CSF release. In the present study, anti-Cdc27, -Emi2, -UbcH10 and -Ube2S antibodies used were all able to immunoprecipitate or immunodeplete their target antigen proteins very efficiently (>90% for immunoprecipitation and >96% for immunodepletion) from CSF extracts ( Figs 1a and 2a ), enabling fairly quantitative assays of the interactions between the respective target proteins. In CSF extracts (before calcium adittion), the core APC/C subunit Cdc27, which is mostly incorporated into the APC/C complexes in Xenopus eggs [33] , [34] , co-immunoprecipitated with another APC/C subunit APC8, with the APC/C coactivator Cdc20 (6% of the total Cdc20 protein, as judged from comparison of the amounts of input Cdc20 and co-precipitated Cdc20, and consistent with previous reports [33] , [34] ), with Emi2 (20%), and with a very small fraction (0.3%) of Ube2S, but not detectably with UbcH10 (similar to previous work [34] ) ( Fig. 2b ). After CSF release (8 min after calcium addition, see Fig. 1b ), Cdc27 (or APC/C) co-precipitated with APC8 and Cdc20 to the same extents as those before CSF release, only little with Emi2 (due to its degradation) and not with UbcH10 (as before CSF release); in contrast to these, however, Cdc27 did co-precipitate with an about fivefold greater fraction (1.5%) of Ube2S than that before CSF release ( Fig. 2b ). Reciprocal Ube2S immunoprecipitation followed by Cdc27 immunoblotting confirmed the fivefold increase in APC/C–Ube2S interactions after CSF release ( Fig. 2c ). Furthermore, in closer analyses, the APC/C–Ube2S interactions turned out to increase immediately (1–2 min) after calcium addition, or concomitantly with the decrease of APC/C–Emi2 interactions and just before the start of cyclin B1 degradation ( Fig. 2d ). Thus, only Ube2S but not UbcH10, although in a very small fraction, seems to increase its interactions with the APC/C on CSF release, inversely correlating with APC/C–Emi2 interactions or Emi2 levels. 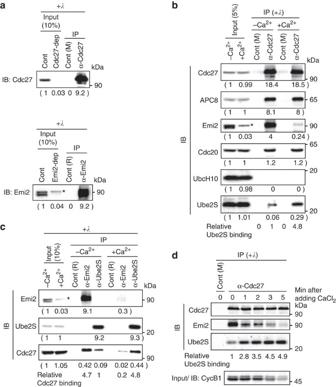Figure 2: APC/C–Ube2S interactions increase after CSF release. (a) Efficient immunoprecititation/immunodepletion of Cdc27 and Emi2 proteins from CSF extracts. For input (10%), both control and Cdc27- or Emi2-immunodepleted extracts were used. Intensities of the blot bands, quantitated using Science Lab 2003 Image Gauge (FUJIFILM), are shown in relative amounts in parentheses. dep, immunodepleted; Cont (M), control mouse IgG; Cont (R), control rabbit IgG. Asterisk, non-Emi2 background protein. (b) CSF extracts either before or 8 min after calcium addition were subjected to Cdc27 immunoprecipitation followed by immunoblotting for the indicated proteins. Relative intensities of the blot bands are shown in parentheses; comparison of the relative intensities of input (5%) and co-immunoprecipitated proteins gives the proportion (see the text) of the co-immunoprecipitate protein in its total protein. Relative Ube2S bindings to Cdc27 (before and after calcium addition) are shown after normalization of (the relative intensity of) co-precipitated Ube2S to immunoprecipitated Cdc27 (although nearly all and equal-amount Cdc27 proteins apparently are immunoprecipitated before and after calcium addition; see also (a)). (c) CSF extracts prepared as in (b) were subjected to either Emi2 or Ube2S immunoprecipitation followed by Cdc27 immunoblotting. Relative intensities of the blot bands are shown in parentheses. Relative Cdc27 bindings to Ube2S are shown after normalization of (the relative intensity of) co-precipitated Cdc27 to immunoprecipitated Ube2S, while those to Emi2 are shown without normalization, which is not applicable in this case, owing to Emi2 degradation after calcium addition (note, however, that similar to Ube2S proteins, nearly all Emi2 proteins present are immunoprecipitated by the antibodies used; see also (a) andFig. 1a). (d) CSF extracts immediately after calcium addition as indicated were subjected to Cdc27 immunoprecipitation followed by either Emi2 or Ube2S immunoblotting. Relative Ube2S bindings to Cdc27, determined as in (b), are also shown; for clarity and conciseness, however, relative intensities of co-precipitated proteins (Emi2 and Ube2S) and immunoprecipitated Cdc27 protein are no longer shown in the figure but are included inSupplementary Fig. 2a. Figure 2: APC/C–Ube2S interactions increase after CSF release. ( a ) Efficient immunoprecititation/immunodepletion of Cdc27 and Emi2 proteins from CSF extracts. For input (10%), both control and Cdc27- or Emi2-immunodepleted extracts were used. Intensities of the blot bands, quantitated using Science Lab 2003 Image Gauge (FUJIFILM), are shown in relative amounts in parentheses. dep, immunodepleted; Cont (M), control mouse IgG; Cont (R), control rabbit IgG. Asterisk, non-Emi2 background protein. ( b ) CSF extracts either before or 8 min after calcium addition were subjected to Cdc27 immunoprecipitation followed by immunoblotting for the indicated proteins. Relative intensities of the blot bands are shown in parentheses; comparison of the relative intensities of input (5%) and co-immunoprecipitated proteins gives the proportion (see the text) of the co-immunoprecipitate protein in its total protein. Relative Ube2S bindings to Cdc27 (before and after calcium addition) are shown after normalization of (the relative intensity of) co-precipitated Ube2S to immunoprecipitated Cdc27 (although nearly all and equal-amount Cdc27 proteins apparently are immunoprecipitated before and after calcium addition; see also ( a )). ( c ) CSF extracts prepared as in ( b ) were subjected to either Emi2 or Ube2S immunoprecipitation followed by Cdc27 immunoblotting. Relative intensities of the blot bands are shown in parentheses. Relative Cdc27 bindings to Ube2S are shown after normalization of (the relative intensity of) co-precipitated Cdc27 to immunoprecipitated Ube2S, while those to Emi2 are shown without normalization, which is not applicable in this case, owing to Emi2 degradation after calcium addition (note, however, that similar to Ube2S proteins, nearly all Emi2 proteins present are immunoprecipitated by the antibodies used; see also ( a ) and Fig. 1a ). ( d ) CSF extracts immediately after calcium addition as indicated were subjected to Cdc27 immunoprecipitation followed by either Emi2 or Ube2S immunoblotting. Relative Ube2S bindings to Cdc27, determined as in ( b ), are also shown; for clarity and conciseness, however, relative intensities of co-precipitated proteins (Emi2 and Ube2S) and immunoprecipitated Cdc27 protein are no longer shown in the figure but are included in Supplementary Fig. 2a . Full size image In the above experiment ( Fig. 2c ), only about 4% of the total Cdc27 protein, as judged by comparison of the amounts of input Cdc27 and co-precipitated Cdc27, was interacting with Emi2 and Ube2S (before and after calcium addition, respectively), indicating that the majority of the APC/C are not complexed with Emi2 or Ube2S. Although the biological significance of this is currently unknown, our findings are rather similar to the observations that the majority (90–95%) of the APC/C are not associated with Cdc20 either, in CSF extracts (while only 6% of Cdc20 itself is complexed with the APC/C; see above) [33] , [34] . Cdc20 is required for APC/C interactions of Ube2S and Emi2 We then asked whether Ube2S could interact with Emi2-associated APC/C or Cdc20-associated APC/C. Consistent with the inverse correlation between the APC/C interactions of Emi2 and Ube2S before and after CSF release, Ube2S failed to be detected in Emi2 immunoprecipitates not only after but also before CSF release (Emi2 is degraded on CSF release) ( Fig. 3a ); vice versa, Emi2 was not detected at all in Ube2S precipitates even before CSF release ( Fig. 3b ). Similar results can be seen in Figs 2c and 3c . Thus, Ube2S does not interact with the APC/C–Emi2 complex nor with APC/C-free Emi2 (which comprises about 80% of the total Emi2 protein before CSF release). In contract, Ube2S co-precipitated with Cdc20, particularly after CSF release, although it did so significantly less efficiently than did Cdc27 and somewhat less efficiently than did Emi2 (before CSF release) ( Fig. 3c ). Interestingly, however, interrupting APC/C–Cdc20 interactions with TAME, a pharmacologic, competitive inhibitor of Cdc20 (refs 35 , 36 ), significantly reduced APC/C interactions of both Ube2S and Emi2 (particularly Emi2) either before or after CSF release ( Fig. 3d ). Immunodepleting Cdc20 had similar but somewhat less significant effects, owing apparently to an inefficient depletion of APC/C-associated Cdc20 ( Supplementary Fig. 3 ). Thus, in CSF extracts, Cdc20 seems to be required, at least in part, for APC/C interactions of both Ube2S and Emi2, perhaps acting to recruit them to the APC/C (see Discussion). 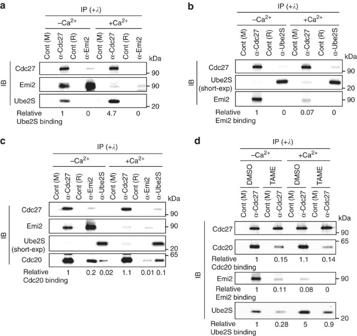Figure 3:Cdc20 is required for bothAPC/C–Emi2andAPC/C–Ube2Sinteractions. (a) CSF extracts either before or 8 min after calcium addition were subjected to either Cdc27 or Emi2 immunoprecipitation followed by Ube2S immunoblotting. (b) CSF extracts prepared as in (a) were subjected to either Cdc27 or Ube2S immunoprecipitation followed by Emi2 immunoblotting. short-exp, a much shorter exposure of the Ube2S blot than that in (a). (c) CSF extracts prepared as in (a) were subjected to immunoprecipitation with the indicated antibodies, followed by Cdc20 immunoblotting. (d) CSF extracts were treated with control solvent dimethyl sulphoxide (DMSO) or TAME (200 μM) for 20 min, incubated with or without calcium for further 8 min and subjected to Cdc27 immunoprecipitation followed by immunoblotting for the indicated proteins. In (a–d), relative Ube2S, Emi2 and Cdc20 bindings to immunoprecipitated proteins were determined as inFig. 2b,c; relative intensities of co-precipitated proteins and immunoprecipitated proteins are included inSupplementary Fig. 2b–e. Figure 3: Cdc20 is required for both APC/C–Emi2 and APC/C–Ube2S interactions. ( a ) CSF extracts either before or 8 min after calcium addition were subjected to either Cdc27 or Emi2 immunoprecipitation followed by Ube2S immunoblotting. ( b ) CSF extracts prepared as in ( a ) were subjected to either Cdc27 or Ube2S immunoprecipitation followed by Emi2 immunoblotting. short-exp, a much shorter exposure of the Ube2S blot than that in ( a ). ( c ) CSF extracts prepared as in ( a ) were subjected to immunoprecipitation with the indicated antibodies, followed by Cdc20 immunoblotting. ( d ) CSF extracts were treated with control solvent dimethyl sulphoxide (DMSO) or TAME (200 μM) for 20 min, incubated with or without calcium for further 8 min and subjected to Cdc27 immunoprecipitation followed by immunoblotting for the indicated proteins. In ( a – d ), relative Ube2S, Emi2 and Cdc20 bindings to immunoprecipitated proteins were determined as in Fig. 2b,c ; relative intensities of co-precipitated proteins and immunoprecipitated proteins are included in Supplementary Fig. 2b–e . Full size image Emi2 directly inhibits APC/C–Ube2S binding via the RL tail We next addressed the important question of how APC/C–Ube2S interactions become increased after CSF release. In earlier results ( Fig. 2d ), APC/C–Ube2S interactions increased immediately after calcium addition, or concomitantly with the disappearance of APC/C–Emi2 interactions. Furthermore, such an increase of APC/C–Ube2S interactions occurred normally even in calcium-treated CSF extracts that were experimentally maintained at Meta-II, but with Emi2 degradation occurring normally ( Supplementary Fig. 4 ). Given these results, the degradation of Emi2 (or the disappearance of APC/C–Emi2 interactions) per se might allow the increase of APC/C–Ube2S interactions on CSF release. Consistent with this idea, merely immunodepleting Emi2 from CSF extracts induced a fivefold increase in APC/C–Ube2S interactions, similar to calcium treatment of the extracts ( Fig. 4a ). Furthermore, treating CSF extracts with okadaic acid (OA), which can dissociate APC/C–Emi2 complexes (without degrading Emi2) by inhibiting Emi2-associated PP2A-B56 phosphatase [19] , [20] , also induced an increase of APC/C–Ube2S interactions, while dissociating the APC/C–Emi2 complexes ( Fig. 4b ). Thus, these results support the idea that the increase of APC/C–Ube2S interactions after CSF release is a result of the disappearance of Emi2 proteins or APC/C–Emi2 interactions on CSF release. 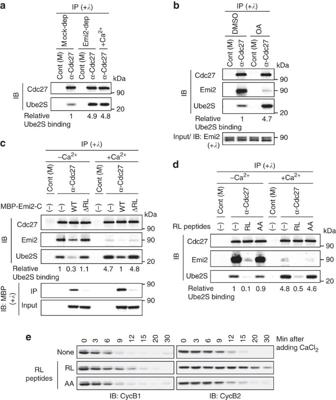Figure 4: Emi2 inhibits APC/C–Ube2S binding via the C-terminal RL tail. (a) CSF extracts mock depleted (using control IgG) or depleted of Emi2 (using anti-Emi2 antibody) were subjected to Cdc27 immunoprecipitation followed by Ube2S immunoblotting. (b) CSF extracts were added with control dimethyl sulphoxide (DMSO) or okadaic acid (OA, 2 μM), and subjected to Cdc27 immunoprecipitation followed by Ube2S or Emi2 immunoblotting. (c) CSF extracts were incubated with MBP–Emi2–C(WT or ΔRL lacking ultimate five amino acids) (0.5 μM), together with or without calcium, for 10 min, and then subjected to Cdc27 immunoprecipitation followed by immunoblotting for the indicated proteins. (d) CSF extracts were incubated with RL tail peptides or AA peptides (1 mM), together with or without calcium, for 10 min, and then analysed as in (c). (e) CSF extracts were added with RL tail or AA peptides concomitantly with calcium, collected at the indicated times and subjected to immunoblotting for cyclin B. Figure 4: Emi2 inhibits APC/C–Ube2S binding via the C-terminal RL tail. ( a ) CSF extracts mock depleted (using control IgG) or depleted of Emi2 (using anti-Emi2 antibody) were subjected to Cdc27 immunoprecipitation followed by Ube2S immunoblotting. ( b ) CSF extracts were added with control dimethyl sulphoxide (DMSO) or okadaic acid (OA, 2 μM), and subjected to Cdc27 immunoprecipitation followed by Ube2S or Emi2 immunoblotting. ( c ) CSF extracts were incubated with MBP–Emi2–C(WT or ΔRL lacking ultimate five amino acids) (0.5 μM), together with or without calcium, for 10 min, and then subjected to Cdc27 immunoprecipitation followed by immunoblotting for the indicated proteins. ( d ) CSF extracts were incubated with RL tail peptides or AA peptides (1 mM), together with or without calcium, for 10 min, and then analysed as in ( c ). ( e ) CSF extracts were added with RL tail or AA peptides concomitantly with calcium, collected at the indicated times and subjected to immunoblotting for cyclin B. Full size image To confirm this idea in a reciprocal way, we also tested whether Emi2 proteins or APC/C–Emi2 interactions, if present even after calcium addition, could inhibit the increase of APC/C–Ube2S interactions. To this end, we added non-degradable, recombinant Emi2 protein (MBP–Emi2–C: Emi2 C-terminal residues 400–651 fused to a maltose-binding protein) and, simultaneously, calcium to CSF extracts. These treatments induced the degradation of endogenous Emi2, instead allowed the binding of MBP–Emi2–C to the APC/C, and inhibited the increase of APC/C–Ube2S interactions ( Fig. 4c ). Furthermore, even without calcium addition, the addition of MBP–Emi2–C reduced the (weak) APC/C–Ube2S interactions in CSF extracts ( Fig. 4c ). Interestingly, in these experiments, however, adding an MBP–Emi2–C variant lacking an Emi2 C-terminal RL tail [MBP–Emi2–C(ΔRL)] failed to inhibit APC/C–Ube2S interactions both before and after calcium addition ( Fig. 4c ). The C-terminal RL tail, named after the ultimate Arg–Leu dipeptide, consists of at least 10 amino acids (see Fig. 5a ) and is essential for Emi2 binding to the APC/C [18] ( Fig. 4c ). Thus, RL tail-mediated Emi2 binding to the APC/C likely interferes with APC/C–Ube2S interactions during CSF arrest, while Emi2 degradation allows the interactions after CSF release. 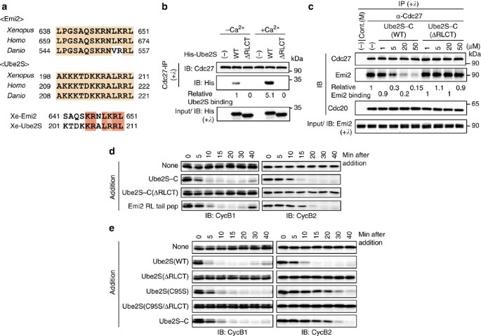Figure 5:An excess of Ube2S can inhibitAPC/C–Emi2interactions via the RL-like C-terminal tail. (a) Alignment of the C-terminal tails of Emi2 and Ube2S proteins from various species. (b) CSF extracts were incubated with His–Ube2S(WT or ΔRLCT lacking ultimate five amino acids) (0.5 μM), together with or without calcium, for 8 min, and then subjected to Cdc27 immunoprecipitation followed by His-tag immunoblotting. (c) CSF extracts were incubated with His–Ube2S–C(WT or ΔRLCT) at the indicated concentrations for 10 min, and subjected to Cdc27 immunoprecipitation followed by immunoblotting for the indicated proteins. (d) CSF extracts were added with His–Ube2S–C(WT or ΔRLCT) (30 μM) or RL tail peptides (1 mM), collected at the indicated times and subjected to cyclin B immunoblotting. (e) CSF extracts were added with the indicated His-Ube2S constructs (10 μM), and analysed as in (d). Figure 5: An excess of Ube2S can inhibit APC/C–Emi2 interactions via the RL-like C-terminal tail. ( a ) Alignment of the C-terminal tails of Emi2 and Ube2S proteins from various species. ( b ) CSF extracts were incubated with His–Ube2S(WT or ΔRLCT lacking ultimate five amino acids) (0.5 μM), together with or without calcium, for 8 min, and then subjected to Cdc27 immunoprecipitation followed by His-tag immunoblotting. ( c ) CSF extracts were incubated with His–Ube2S–C(WT or ΔRLCT) at the indicated concentrations for 10 min, and subjected to Cdc27 immunoprecipitation followed by immunoblotting for the indicated proteins. ( d ) CSF extracts were added with His–Ube2S–C(WT or ΔRLCT) (30 μM) or RL tail peptides (1 mM), collected at the indicated times and subjected to cyclin B immunoblotting. ( e ) CSF extracts were added with the indicated His-Ube2S constructs (10 μM), and analysed as in ( d ). Full size image These results suggest either that Emi2 bound to the APC/C (via the RL tail) somehow inhibits APC/C–Ube2S interactions or, more likely, that APC/C binding of the RL tail itself inhibits Ube2S from binding to the APC/C. To test the latter possibility directly, we added an excess of synthetic RL tail peptides (residues 636–651, see Fig. 5a ) and, simultaneously, calcium to CSF extracts. The RL tail peptides, but not its ultimate dipeptide RL→AA peptides, strongly inhibited the increase of APC/C–Ube2S interactions after CSF release (as well as inhibiting the weak APC/C–Ube2S interactions during CSF arrest and also APC/C–Emi2 interactions) ( Fig. 4d ). Because RL tail peptides, but not AA peptides, can directly bind to the APC/C [18] , [19] , these results strongly suggest that APC/C binding of the Emi2 RL tail can by itself inhibit Ube2S binding to the APC/C, thereby impairing Ube2S function and, hence, APC/C activity. Consistent with this, adding RL tail (but not AA) peptides, together with calcium, to CSF extracts was able to delay the degradation of cyclin B ( Fig. 4e ), similar to immunodepletion of Ube2S ( Fig. 1c ). An excess of Ube2S can disrupt APC/C–Emi2 binding Reportedly, the C-terminal tail of Ube2S is important for the activity of Ube2S towards the APC/C and is required for Ube2S to bind to the APC/C coactivator Cdh1 (refs 27 , 28 ). Interestingly, this Ube2S C-terminal tail is well conserved and is very similar to the Emi2 RL tail ( Fig. 5a ). Given this similarity as well as the ability of APC/C–Ube2S binding to be inhibited by the Emi2 RL tail ( Fig. 4c–e ), the Ube2S C-terminal tail, which herein we refer to as RLCT for Emi2 RL-like C-terminal tail, may be a Ube2S’s APC/C binding site and could be competed with by the Emi2 RL tail. Consistently, while exogenously introduced, His 6 -tagged wild-type Ube2S [His–Ube2S(WT)], like endogenous Ube2S ( Fig. 2 ), could bind to the APC/C fivefold more strongly after CSF release than before, a His–Ube2S mutant lacking the RLCT [His–Ube2S(ΔRLCT)] could not bind to the APC/C at all ( Fig. 5b ). Thus, RLCT is essential for Ube2S to bind to the APC/C both before and after CSF release. We then asked whether an excess of RLCT could affect APC/C–Emi2 interactions. As shown in Fig. 5c , adding His 6 -tagged Ube2S C-terminal fragments (residues 162–211) (His–Ube2S–C), but not those lacking the RLCT [His–Ube2S–C(ΔRLCT)], to CSF extracts disrupted APC/C–Emi2 interactions in a dose-dependent manner, whereas it could not affect APC/C–Cdc20 interactions (as control) at all. Under the present conditions, as high as 20–50 μM His–Ube2S–C protein was required to efficiently (>80%) disrupt the APC/C–Emi2 interactions ( Fig. 5c ); however, this perhaps reflected the much weaker APC/C binding of endogenous Ube2S than that of Emi2 (despite its much higher concentration (220 nM) than that of Emi2 (15 nM; ref. 17 ) in CSF extracts) ( Fig. 2c ). Regardless, adding His–Ube2S–C but not His–Ube2S–C(ΔRLCT) (30 μM) to CSF extracts readily induced cyclin B degradation (perhaps mediated by multiple monoubiquitination by UbcH10 (ref. 30 )) even without calcium addition, similar to the addition of Emi2 RL tail peptides ( Fig. 5d ). Furthermore, most probably because of its intact E2 enzymatic activity as well as its ability to disrupt APC/C–Emi2 interactions, full-length His–Ube2S(WT) (10 μM), but not His–Ube2S(ΔRLCT), could induce cyclin B degradation significantly even more rapidly than His–Ube2S–C and His–Ube2S(C95S), which are both catalytically inactive [28] ( Fig. 5e ). Thus, in its excess, Ube2S can competitively inhibit APC/C–Emi2 interactions via APC/C binding of its RLCT, thereby causing APC/C activation and, hence, cyclin B degradation without calcium addition. Altogether ( Figs 4 and 5 ), these results strongly suggest that, before CSF release, Emi2 competitively inhibits Ube2S binding to the APC/C by APC/C binding of its RL tail, but, on CSF release, degradation of Emi2 relieves its competitive inhibition of the (RLCT-mediated) APC/C–Ube2S binding, thereby contributing significantly to APC/C activation at fertilization. In this context, we note that the amount (concentration) of the APC/C–Ube2S complexes after CSF release is very close to that of the APC/C–Emi2 complexes before CSF release ( Fig. 2c ); they are both about 3 nM, given the concentrations of the total Ube2S protein (220 nM) and Emi2 protein (15 nM), as well as the proportions of APC/C-associated Ube2S (1.5% of the total Ube2S protein, after CSF release) and Emi2 (20%, before CSF release), in CSF extracts. Interestingly, it has recently been shown that Emi1, a somatic paralog of Emi2, can competitively inhibit APC/C–Ube2S binding in vitro [31] . Emi2 and Ube2S bind to APC10 via their C-terminal tails Given our results, Emi2 and Ube2S could bind to the same site(s) of the APC/C via their similar C-terminal tails. In vertebrates, the APC/C consists of as many as 14 different subunits; among these subunits, seven (Cdc27(APC3), APC6, APC7, APC8(Cdc23), Cdc26(APC12), APC13 and APC16) are located in the arc lamp domain, three (APC2, APC10 and APC11) in the catalytic core domain and four (APC1, APC4, APC5 and APC15) in the platform domain of the APC/C [21] , [22] . A previous study showed that recombinant Emi2 protein can bind to three APC/C subunits, APC6, APC10 and APC11, that were expressed in rabbit reticulocyte lysates [17] , although it remained unclear whether these bindings depended on the Emi2 RL tail. We first examined, by pulldown assays, whether MBP–Emi2–C could bind, via the RL tail, to any of the 14 different APC/C subunits individually expressed in similar rabbit reticulocyte lysates. As shown in Fig. 6a ; Supplementary Fig. 5a , MBP–Emi2–C(WT) was able to bind to (Myc 3 -tagged) Cdc27, APC8 and APC10, but not to the other APC/C subunits, several fold more strongly than MBP–Emi2–C(ΔRL) and MBP alone. Thus, in our study, APC6 and APC11, which (besides APC10) were reported to bind Emi2 (ref. 17 ), failed to bind Emi2 in an RL tail-dependent manner (they seemed to bind Emi2 rather non-specifically or, at least, in an RL tail-independent manner; Fig. 6a ; Supplementary Fig. 5a ). We then tested whether His–Ube2S protein could bind, via the RLCT, to any APC/C subunit(s) similarly expressed in reticulocyte lysates. His–Ube2S(WT) bound to (Myc 3 -tagged) Cdc27, APC8, APC10 and APC16, but not to the other APC/C subunits, significantly more strongly than His–Ube2S(ΔRLCT) and beads alone ( Fig. 6b ; Supplementary Fig. 5b ). Thus, Emi2 and Ube2S seemed to bind commonly to three APC/C subunits, that is, Cdc27, APC8 and APC10, via their C-terminal tails when the subunits were expressed in rabbit reticulocyte lysates. 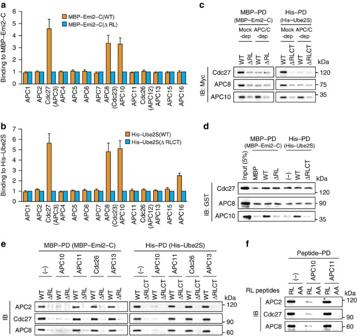Figure 6: Emi2 and Ube2S bind to the APC10 subunit of the APC/C. (a) Various Myc3-tagged APC/C subunits individually expressed in rabbit reticulocyte lysates were subjected to pulldown assays using either MBP alone, MBP–Emi2–C(WT) or MBP–Emi2–C(ΔRL), each coupled to beads, and after Myc immunoblotting, quantitated using Science Lab 2003 Image Gauge (FUJIFILM). For each APC/C subunit, binding to MBP–Emi2–C(WT) relative to that to MBP–Emi2–C(ΔRL) is shown (with mean±s.d.,n=4). Original immunoblotting data are presented inSupplementary Fig. 5a, which also includes binding to MBP alone. (b) Similar experiments to (a) except that pulldown assays were performed using either His-Ube2S(WT) or His-Ube2S(ΔRLCT), each coupled to beads, or beads alone (−). For each APC/C subunit, binding to His-Ube2S(WT) relative to that to His-Ube2S(ΔRLCT) is shown (mean±s.d.,n=4). Original immunoblotting data are presented inSupplementary Fig. 5b, which also includes binding to beads only. (c) The indicated Myc3-tagged APC/C subunits were expressed in reticulocyte lysates mock depleted or depleted of endogenous APC/C complexes, subjected to pulldown assays using either MBP–Emi2–C(WT or ΔRL) or His-Ube2S(WT or ΔRLCT), and analysed by Myc immunoblotting. (d) The indicated GST-APC/C subunit proteins were subjected to pulldown assaysin vitrousing either MBP–Emi2–C(WT or ΔRL) or His-Ube2S(WT or ΔRLCT), and analysed by GST-tag immunoblotting. (e) Reticulocyte lysates were added with the indicated GST-APC/C subunit proteins (20 μM) or buffer alone (−), subjected to pulldown assays using either MBP–Emi2–C(WT or ΔRL) or His-Ube2S(WT or ΔRLCT), and immunoblotted for endogenous APC/C subunit proteins. (f) Reticulocyte lysates added with GST-APC10 or GST-APC11 (20 μM) were subjected to pulldown assays using either RL tail or AA peptides, each coupled to beads, and then immunoblotted for APC/C subunit proteins. Figure 6: Emi2 and Ube2S bind to the APC10 subunit of the APC/C. ( a ) Various Myc 3 -tagged APC/C subunits individually expressed in rabbit reticulocyte lysates were subjected to pulldown assays using either MBP alone, MBP–Emi2–C(WT) or MBP–Emi2–C(ΔRL), each coupled to beads, and after Myc immunoblotting, quantitated using Science Lab 2003 Image Gauge (FUJIFILM). For each APC/C subunit, binding to MBP–Emi2–C(WT) relative to that to MBP–Emi2–C(ΔRL) is shown (with mean±s.d., n =4). Original immunoblotting data are presented in Supplementary Fig. 5a , which also includes binding to MBP alone. ( b ) Similar experiments to ( a ) except that pulldown assays were performed using either His-Ube2S(WT) or His-Ube2S(ΔRLCT), each coupled to beads, or beads alone (−). For each APC/C subunit, binding to His-Ube2S(WT) relative to that to His-Ube2S(ΔRLCT) is shown (mean±s.d., n =4). Original immunoblotting data are presented in Supplementary Fig. 5b , which also includes binding to beads only. ( c ) The indicated Myc 3 -tagged APC/C subunits were expressed in reticulocyte lysates mock depleted or depleted of endogenous APC/C complexes, subjected to pulldown assays using either MBP–Emi2–C(WT or ΔRL) or His-Ube2S(WT or ΔRLCT), and analysed by Myc immunoblotting. ( d ) The indicated GST-APC/C subunit proteins were subjected to pulldown assays in vitro using either MBP–Emi2–C(WT or ΔRL) or His-Ube2S(WT or ΔRLCT), and analysed by GST-tag immunoblotting. ( e ) Reticulocyte lysates were added with the indicated GST-APC/C subunit proteins (20 μM) or buffer alone (−), subjected to pulldown assays using either MBP–Emi2–C(WT or ΔRL) or His-Ube2S(WT or ΔRLCT), and immunoblotted for endogenous APC/C subunit proteins. ( f ) Reticulocyte lysates added with GST-APC10 or GST-APC11 (20 μM) were subjected to pulldown assays using either RL tail or AA peptides, each coupled to beads, and then immunoblotted for APC/C subunit proteins. Full size image Surprisingly, during the course of these experiments, however, we found that rabbit reticulocyte lysates contained a significant amount of endogenous APC/C complexes, which were able to specifically bind both MBP–Emi2–C(WT) and His–Ube2S(WT), but not their C-terminal-lacking mutants ( Supplementary Fig. 5c ). Furthermore, and notably, a significant fraction (5–10%) of Myc-Cdc27 and Myc-APC8, but not of Myc-APC10, was found to be incorporated into the endogenous APC/C complexes ( Supplementary Fig. 5d ). Given these results, the bindings of Myc-Cdc27 and Myc-APC8, but not of Myc-APC10, with both MBP–Emi2–C(WT) and His–Ube2S(WT) ( Fig. 6a,b ) could have been indirect (or endogenous APC/C-mediated) bindings, owing to their incorporations into the endogenous APC/C complexes. To test this possibility, we utilized reticulocyte lysates that were immunodepleted of endogenous APC/C complexes (using both anti-Cdc27 and anti-APC2 antibodies; Supplementary Fig. 5e ). In such lysates but not in mock-depleted lysates, both Myc-Cdc27 and Myc-APC8, but not Myc-APC10, failed to significantly bind either MBP–Emi2–C(WT) or His–Ube2S(WT) ( Fig. 6c ). Thus, only APC10, but not Cdc27 or APC8, can specifically bind both Emi2 and Ube2S at the C-terminal tails even without endogenous APC/C complexes, suggesting a direct binding of only APC10 to Emi2(WT) and Ube2S(WT). Indeed, in in vitro binding assays, glutathione S -transferase (GST)-fused APC10 protein, but not Cdc27 or APC8 proteins, could bind both MBP–Emi2–C(WT) and His–Ube2S(WT) significantly more strongly than their C-terminal-lacking mutants ( Fig. 6d ). Thus, APC10 can directly bind both Emi2 and Ube2S at the C-terminal tails. These results suggested that, among all 14 different APC/C subunits, APC10, a catalytic core subunit, is the only common Emi2/Ube2S-binding site of the APC/C. To confirm this, we also asked whether an excess of APC10 protein could competitively inhibit the binding of endogenous APC/C complexes with Emi2 and Ube2S in reticulocyte lysates. Adding GST-APC10 (20 μM), but not similar-sized control GST-APC/C subunits (APC11, Cdc26 and APC13) at the same concentrations, to reticulocyte lysates specifically inhibited endogenous APC/C complexes from binding MBP–Emi2–C(WT) and His–Ube2S(WT) ( Fig. 6e ). The inability of an excess of GST-APC11 protein to competitively inhibit APC/C binding to Ube2S is particularly interesting because APC11, another catalytic core subunit, is thought to bind E2 enzymes generally [3] , [22] ; however, this inability is consistent with APC11 being all unable to bind Ube2S ( Fig. 6b ; Supplementary Fig. 5b ). In reticulocyte lysates, adding GST-APC10, but not GST-APC11, also inhibited the binding of endogenous APC/C complexes with RL tail peptides coupled to beads ( Fig. 6f ), indicating that, in Fig. 6e , APC10 competed with the APC/C complexes for binding Emi2 (and Ube2S) at the C-terminal tails. Taken together, these results strongly suggest that Emi2 and Ube2S both bind to the APC/C catalytic core subunit APC10 via their C-terminal tails. Our results clearly show that Ube2S and UbcH10 play a significant role for the degradation of both cyclin B1 and B2 and, hence, also for the subsequent nuclear envelope formation on CSF release of unfertilized Xenopus egg extracts. However, depletion of Ube2S alone cannot strongly inhibit cyclin B1 degradation, whereas co-depletion of Ube2S and UbcH10 can do so. This might be because UbcH10 (and possibly also UbcH5) can catalyse multiple monoubiquitination of cyclin B1 (ref. 30 ). Interestingly, however, our results differ from those of Dimova et al. [30] showing that single depletion of either UbcH10 or Ube2S has no detectable effects on cyclin B1(WT) degradation in mitotically arrested Xenopus egg extracts (despite the proposed sufficiency of UbcH10-catalysed multiple monoubiquitination for cyclin B1 degradation). This apparent difference might be owing to the difference between the natures of egg extracts used by the two groups (calcium-treated meiotic CSF extracts vs non-degradable cyclin B-treated mitotic extracts) or, alternatively, owing to the difference between the intervals of kinetics employed for analysis of cyclin B1 degradation (a few minutes vs 15 min). Regardless, our results indicate that Ube2S or its ubiquitin chain-elongating activity is required for the rapid degradation of both cyclin B1 and B2, and thus plays a physiologically important role on fertilization of Xenopus eggs ( Fig. 7 ). Given our results and those in Drosophila cells [27] , Ube2S may play a role in cyclin B degradation more generally during normal mitosis than previously thought, that is, than only during recovery from the spindle checkpoint as in human cells [26] . 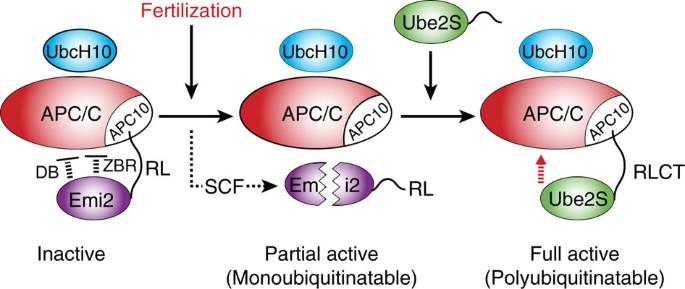Figure 7:Model for the regulation of APC/C activity before and after fertilization ofXenopuseggs. The APC/C activity is inhibited by RL tail-mediated Emi2 binding to APC10 (hence, by the action of the D-box and the ZBR and also by the competitive inhibition of APC/C–Ube2S binding) before fertilization, becomes partially active (or monoubiquitinatable) due to both (SCFβ-TrCP-dependent) Emi2 degradation and UbcH10 activity on fertilization, and then becomes fully active (or polyubiquitinatable) by RLCT-mediated Ube2S binding to APC10. The ‘partial’ to ‘full’ transition of the APC/C activity at fertilization is very quick because Ube2S binding to the APC/C occurs instantaneously on Emi2 degradation. Although not shown in the figure, the APC/C coactivator Cdc20 is required, at least in part, for the binding of Emi2 and Ube2S to the APC/C. InXenopuseggs, the binding site of UbcH10 in the APC/C is currently unknown. Figure 7: Model for the regulation of APC/C activity before and after fertilization of Xenopus eggs. The APC/C activity is inhibited by RL tail-mediated Emi2 binding to APC10 (hence, by the action of the D-box and the ZBR and also by the competitive inhibition of APC/C–Ube2S binding) before fertilization, becomes partially active (or monoubiquitinatable) due to both (SCF β-TrCP -dependent) Emi2 degradation and UbcH10 activity on fertilization, and then becomes fully active (or polyubiquitinatable) by RLCT-mediated Ube2S binding to APC10. The ‘partial’ to ‘full’ transition of the APC/C activity at fertilization is very quick because Ube2S binding to the APC/C occurs instantaneously on Emi2 degradation. Although not shown in the figure, the APC/C coactivator Cdc20 is required, at least in part, for the binding of Emi2 and Ube2S to the APC/C. In Xenopus eggs, the binding site of UbcH10 in the APC/C is currently unknown. Full size image Interestingly, our results show that APC/C–Ube2S interactions increase several fold on CSF release, inversely correlating with APC/C–Emi2 interactions, and that Cdc20 (or its interaction with the APC/C) is required, at least in part, for APC/C interactions of both Ube2S and Emi2. Normally, Cdc20 directly interacts with D-box degron-containing proteins (mostly APC/C substrates) and recruits them to the APC/C [21] , [37] . Interestingly, both Emi2 and Ube2S harbour D-box motifs and are potential APC/C substrates under certain conditions [16] , [27] . Therefore, our results would seem to suggest that, in CSF extracts, Cdc20 initially interacts with either Emi2 or Ube2S, and thereby facilitates their binding to the APC/C, resulting in the formation of Cdc20–APC/C–Emi2 and Cdc20–APC/C–Ube2S ternary complexes mainly before and after CSF release, respectively. However, Cdc20 could also function to maintain APC/C binding of Emi2 and Ube2S, for example, by changing the conformation of the APC/C [38] , because we also observed the importance of APC/C-associated Cdc20 for sustained APC/C binding of Emi2 and Ube2S ( Supplementary Fig. 3 ). Importantly, our study shows that, during CSF arrest, Emi2 directly inhibits Ube2S binding to the APC/C by APC/C binding of its C-terminal RL tail, but, on CSF release (or fertilization), degradation of Emi2 relieves its inhibition of the APC/C–Ube2S binding, thereby enabling the rapid degradation of cyclin B1 and B2 ( Fig. 7 ). Interestingly, Ube2S harbours an RL-like C-terminal tail (RLCT), and, in its excess, RLCT can inhibit APC/C–Emi2 interactions even during CSF arrest. Thus, most likely, Emi2 and Ube2 compete with each other for APC/C binding via their similar C-terminal tails. Somewhat curiously, only a small fraction of Emi2 and Ube2S, particularly of Ube2S, binds to the APC/C via their C-terminal tails; however, this might be due to the (not yet proven) catalytic-like action (for Emi2) and the catalytic action (for Ube2S) on the APC/C [17] , [39] . Furthermore, Ube2S, although its concentration in CSF extracts is >10-fold higher than that of Emi2, cannot efficiently bind to the APC/C in the presence of Emi2. The reason for this is currently unknown, but might be because the RLCT of Ube2S lacks such a neighbouring element as the ZBR of Emi2, which contributes to APC/C–Emi2 binding, while directly inhibiting APC/C activity [17] , [18] . Yet, the high concentration of Ube2S (220 nM), which is greater even than that of the APC/C (80 nM, considering two copies of Cdc27 per APC/C complex [17] , [21] ), might be required for the instantaneous APC/C binding of Ube2S on Emi2 degradation. At all events, our study demonstrates an important role for Emi2 binding to the APC/C, that is, a competitive inhibition of APC/C–Ube2S binding, in APC/C regulation, in addition to the well-established role for it in directly inhibiting APC/C activity, albeit via the action of ZBR [19] , [33] . Furthermore, Emi2 degradation plays a significant role in promoting Ube2S binding to the APC/C, in addition to the role in liberating the APC/C from inhibition by the Emi2 ZBR. Thus, APC/C binding, as well as degradation, of Emi2 has a novel (and dual) role in regulating APC/C activity, thereby robustly controlling CSF arrest and release (or fertilization) of Xenopus eggs ( Fig. 7 ). At the nearly final step of this work, Wang and Kirschner [31] reported that the C-terminal tail of Emi1, a somatic paralog of Emi2 (refs 22 , 40 ), can competitively inhibit Ube2S binding to the APC/C in vitro , and that Emi1 and Ube2S both bind to the APC/C catalytic core subunit APC2. Our study establishes that Emi2 inhibits APC/C–Ube2S binding in a manner similar to Emi1 but under physiological conditions, or during CSF arrest of Xenopus eggs, and that Emi2 degradation causes APC/C–Ube2S binding to activate the APC/C under physiological conditions, or at fertilization. In contrast to the results of Wang and Kirschner [31] , however, our study demonstrates that Emi2 and Ube2S both bind to the APC10 subunit, not APC2, of the APC/C. The reason for this apparent discrepancy is currently unknown. However, on the basis of the interaction between the cullin subunit (of SCF ubiquitin ligase) and the E2 enzyme Cdc34 (ref. 41 ), the above authors [31] suspected APC2, the cullin subunit of the APC/C [21] , to be a Ube2S (and Emi1)-binding site of the APC/C, eventually showing that both Ube2S and Emi1 can interact with APC2 ectopically expressed in rabbit reticulocyte lysates. Unexpectedly, in our study, however, rabbit reticulocyte lysates do contain a significant amount of endogenous APC/C complexes ( Supplementary Fig. 5c ), and although Emi2 and Ube2S can both readily co-precipitate with endogenous APC2 (as well as other APC/C subunits) associated with the endogenous APC/C complexes ( Fig. 6e ; Supplementary Fig. 5c ), they cannot bind at all to ectopically expressed, endogenous APC/C complex-free APC2 ( Fig. 6a,b ). Thus, in the Wang and Kirschner paper [31] , the APC2 protein detected with anti-APC2 antibody and thought to be bound directly to Emi1 and Ube2S might be endogenous APC2 that is complexed with the endogenous APC/C, which perhaps binds Emi1/Ube2S via another APC/C subunit(s), probably APC10. Indeed, in our study, among all the known 14 APC/C subunits tested, only APC10, a catalytic core subunit, can directly bind both Emi2 and Ube2S at the C-terminal tails. Thus, most likely, Emi2 and Ube2S commonly bind to the APC10 subunit of the APC/C, which is not inconsistent with the recently reported EM structure of human APC/C Cdh1 -Emi1, in which the C terminus of Emi1 interacts with the catalytic core and/or platform regions of the APC/C [42] . APC10, a catalytic core subunit with APC/C substrate recognition [43] , [44] , is also required for processivity of polyubiquitination of APC/C substrates [38] , [45] , [46] . Our results suggest that this requirement of APC10 for processivity can occur because APC10 now appears to be the factor that binds Ube2S, a major processivity E2 enzyme for the APC/C in higher eukaryotes [26] , [27] , [28] . To summarize, our results and those of Wang and Kirschner [31] demonstrate that an Emi1/Emi2 family of proteins, unlike other APC/C inhibitors [3] , plays a novel, important role in regulating APC/C activity, that is, a competitive inhibition of APC/C–Ube2S binding. In addition, our results reveal that Emi2 degradation triggers APC/C–Ube2S binding at fertilization to activate the APC/C. Given these results, it will be interesting to know whether, in somatic cells, Ube2S begins to interact with the APC/C at prometaphase of the cell cycle, a time when Emi1 becomes degraded, leading to APC/C activation [47] , [48] . Biochemical reagents Sources of major biochemical reagents were as follows: λ phosphatase (NEB); TAME (SIGMA); OA (Wako); Dynabeads protein G (Invitrogen); NHS-activated Sepharose 4 Fast Flow beads (GE Healthcare); maltose-bound beads (NEB); Nickel-agarose beads (Nacalai); rabbit reticulocyte lysates (Promega). CSF extracts CSF extracts were prepared from unfertilized Xenopus eggs and treated with 600 μM CaCl 2 to induce a release from CSF arrest [18] . In some cases, demembranated sperm nuclei (final 2,500 nuclei per microlitre) were added to the CSF extracts and stained with Hoechst 33342 (ref. 49 ). Experiments using Xenopus were approved by the Animal Care and Use Committee, Kyushu University. cDNAs and in vitro transcription/translation The complementary DNA (cDNA) for Xenopus Emi2 was described previously (AF450296 in the Entrez Nucleotide database) [8] . The cDNAs for Xenopus UbcH10(UbcX), Ube2S, Cdc27(APC3), APC4, APC5, APC6, APC7, APC8(Cdc23), APC10, APC11, Cdc26(APC12) and APC13 were isolated by PCR from a Xenopus ovarian cDNA library, whereas those for human APC1, APC2, APC15 and APC16 were from a HeLa cell cDNA library. The cDNAs were subcloned into the N-terminally Myc 3 -tagged pT7G (UKII−) transcription vector [8] . Point mutations and deletions were generated by site-directed mutagenesis using appropriate primers (shown in Supplementary Table 1 ) and a Quick Change Kit (Stratagene). In vitro transcription of the cDNAs was performed essentially as we described earlier [19] , whereas in vitro translation was performed in 30 μl of rabbit reticulocyte lysates supplemented with 0.4–0.8 μg of in vitro transcribed mRNA [50] . Recombinant proteins and synthetic peptides His 6 -tagged Ube2S proteins (WT or ΔRLCT lacking ultimate five amino-acid residues), MBP-fused Emi2 C-terminal fragments (WT or ΔRL lacking ultimate five amino-acid residues) and GST-fused APC/C subunit proteins were bacterially expressed and purified using nickel-agarose beads (Nacalai), maltose-bound beads (NEB) and glutathione-Sepharose 4B beads (GE Healthcare), respectively, according to the manufacturers’ instructions. Synthetic RL tail peptides and its RL→AA peptides, each consisting of 16 amino acids, were those we described previously [18] . Antibodies and immunoblotting Antibodies against His 6 -tagged, full-length Xenopus UbcH10 and Ube2S proteins were raised in rabbits and purified using nickel-agarose beads (Nacalai) according to the manufacturer’s instructions, whereas antibodies against Xenopus Emi2 and cyclin B1 and B2 were those we described previously [8] , [18] . Sources of other antibodies used were as follows: anti-Myc-epitope (Cell Signaling; 2276S); anti-His (MBL; M136-3); anti-MBP (NEB; E8032S); anti-GST (Abcam; ab9085); anti-Cdc27 (BD Biosciences; 610455); anti-APC8/Cdc23 (Abcam; ab72206); anti-Cdc20 (gift from H. Yamano); anti-APC2 (SIGMA; A4358); anti-APC1 (Abcam; ab133397); anti-APC10 (Abcam; ab126204). Immunoblotting was performed essentially as we described previously [8] , [19] ; dilutions of the respective antibodies are presented in Supplementary Table 2 . For immunoblotting of co-immunoprecipitated Cdc20 or Ube2S proteins, however, immunoprecipitates were treated with a high-salt washing buffer containing 500 mM NaCl (instead of 5 mM KCl in the low-salt washing buffer described below), and the supernatants (containing Cdc20 or Ube2S but not antibodies) were subjected to immunoblotting (otherwise Cdc20 and Ube2S co-migrated, on SDS–PAGE, with the heavy and light chains, respectively, of the co-precipitated antibodies, and ran aberrantly). Furthermore, for immunoblotting of proteins newly synthesized in reticulocyte lysates, immunoprecipitates were transferred to a fresh tube before subjecting to immunoblotting, because a significant fraction of the newly synthesized (particularly APC10) proteins tended to stick to the original tube. Full scans of all immunoblots are included in Supplementary Figs 6–12 . Immunoprecipitation and immunodepletion For immunoprecipitation, routinely 30 μl of CSF extracts or rabbit reticulocyte lysates (Promega) were mixed with 2–4 μg of specified antibodies coupled to 10–20 μl of a slurry of protein G-conjugated Dynabeads (Invitrogen), and incubated for 30 min at 4 °C with tapping at every 5 min intervals. CSF extracts immediately after calcium addition ( Fig. 2d ) were added with EGTA (final 30 mM) and MG262 (200 μM) before immunoprecipitation. The immunoprecipitates were freed of extracts or lysates nearly completely by centrifugation and magnetic-stand treatment, which were repeated once again, washed twice with 100 μl of a low-salt washing buffer (20 mM Tris-HCl, pH7.5, 5 mM KCl, 5 mM 6DAP, 1 mM DTT, 2 mM NaF, 1 μM OA, 20 μM leupeptin, 2 μM pepstatin, 10 μg μl −1 aprotinin, 400 μM PMSF and 0.1% Tween 20), treated or not treated with 1 μg of λ phosphatase [50] , and then subjected to immunoblotting. For immunodepletion, routinely 30 μl of CSF extracts or reticulocyte lysates were treated with specified antibodies coupled to protein G-conjugated Dynabeads as described above (except that the incubation time was 20 min), and the supernatants were treated once again with the same antibodies and then served as immunodepleted extracts or lysates. Pulldown assays For pulldown assays, routinely 30 μl of rabbit reticulocyte lysates were incubated with 0.5 μg of His–Ube2S(WT or ΔRLCT) protein coupled to 5 μl of a slurry of nickel-agarose beads (Nacalai), with 2 μg of MBP–Emi2–C(WT or ΔRL) protein coupled to 10 μl of a slurry of maltose-bound beads (NEB) or with 30 μg of RL tail (WT or AA) peptides coupled to 10 μl of a slurry of NHS-beads (GE Healthcare) for 30 min at 4 °C. The beads were freed of lysates nearly completely by two rounds of brief centrifugation (and removal of supernatants), washed twice with 100 μl of a low-salt washing buffer (see above) and then subjected to immunoblotting. How to cite this article: Sako, K. et al. Emi2 mediates meiotic MII arrest by competitively inhibiting the binding of Ube2S to the APC/C. Nat. Commun. 5:3667 doi: 10.1038/ncomms4667 (2014).